Marine protected area improves yield without disadvantaging fishers Potential fishery benefits of Marine Protected Areas (MPAs) are widely acknowledged, yet seldom demonstrated, as fishery data series that straddle MPA establishment are seldom available. Here we postulate, based on a 15-year time series of nation-wide, spatially referenced catch and effort data, that the establishment of the Goukamma MPA (18 km alongshore; 40 km 2 ) benefited the adjacent fishery for roman ( Chrysoblephus laticeps ), a South African endemic seabream. Roman-directed catch-per-unit-effort (CPUE) in the vicinity of the new MPA immediately increased, contradicting trends across this species’ distribution. The increase continued after 5 years, the time lag expected for larval export, effectively doubling the pre-MPA CPUE after 10 years. We find no indication that establishing the MPA caused a systematic drop in total catch or increased travel distances for the fleet. Our results provide rare empirical evidence of rapidly increasing catch rates after MPA implementation without measurable disadvantages for fishers. The effects of no-take Marine Protected Areas (MPAs) on exploited fish populations are now well studied [1] , [2] , yet their impacts on fishery dynamics remain poorly documented and their benefits to fishers questionable [3] , [4] , [5] , [6] . To be beneficial to fisheries, MPAs need to be designed to protect spawning stocks and to boost fishery yield via net emigration of adult fish (spillover) and the export of larvae. In theory, these processes should result in a two-step improvement for the fishery, an immediate, steady increase in catch rates in adjacent fishing areas due to net export of adult fishes as a result of the increasing biomass gradient, and an amplification of this effect after a lag phase equivalent to or longer than the age-at-recruitment. The cumulative effect needs to outweigh the possible short-term reduction of fisher’s profits because of increased travel times and decreased catch-per-unit-effort (CPUE) when fishing is displaced [7] , within an economically acceptable time frame. The magnitude and timing of MPA effects are functions of fishing intensity, stock status, species biology, and size and location of the reserve. The application of MPAs in fishery management remains controversial, because few empirical studies have evaluated the effect of closures on fishery yield [7] and fleet behaviour [8] ; therefore, sustained benefits for fishers can seldom be clearly demonstrated [3] . Spillover and larval export effects are difficult to detect in fishery data. Shifts in fishing effort and catchability, fluctuations in population abundance, market-related factors and environmental change all influence catch rates and may confound potential effects of area closure. Furthermore, spatially referenced time series of catch and effort data seldom straddle the implementation dates of MPAs, and when they do, observed changes can seldom be ascribed unequivocally to reserve effects because of the difficulty of finding suitable reference sites [4] , [9] . We examined total catches and CPUE for possible effects of the implementation of the Goukamma MPA on the catch of roman ( Chrysoblephus laticeps ), a protogynous seabream endemic to South Africa’s warm-temperate coast. Roman occur as a single, well-mixed population [10] , which is exploited throughout its range by the South African boat-based, multi-species linefishery, for which spatially referenced, species- and boat-specific catch reporting has been mandatory since 1985 ( Fig. 1a ). The Goukamma MPA (18 km alongshore; 40 km 2 ) is in the centre of the roman distribution. The MPA was implemented in 1990 and prohibits all boat-based fishing. The fishery for roman around Goukamma presents a rare opportunity to study the MPA effect because catch and effort data on roman are available continuously throughout the range of this species from well before and after the reserve was established. We examined the time series up to the year 2000, when drastic, nation-wide cuts in effort were implemented to rebuild depleted linefish stocks. The linefishery was fairly stable in this period in terms of participants, total catch and effort. The low initial stock level, suggested by a decrease of CPUE by 83 to 95% compared with historical values [11] , and the high degree of residency of roman [12] , [13] provided for a big recovery potential for fish density inside the MPA and for catches within the area of possible influence of spillover and larval dispersal. 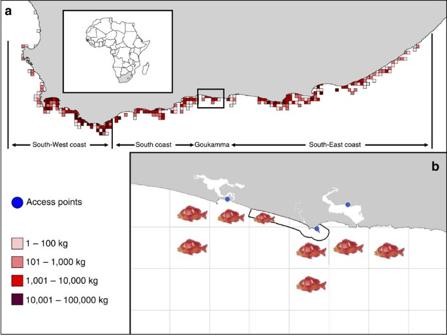Figure 1: Roman landings per coastal area throughout the range of the species. (a) Four areas (South-West coast, South coast, Goukamma and South-East coast) along the coast of South Africa (insert) for which roman catches were reported by the boat-based commercial linefishery. Total landings of roman for the period 1985–2000 per 5 × 5 nautical mile grid cell are shown. (b) Goukamma area with boundaries of the MPA and access points (blue circles) for the local fishery. Grid cells where roman catches were reported are indicated. Figure 1: Roman landings per coastal area throughout the range of the species. ( a ) Four areas (South-West coast, South coast, Goukamma and South-East coast) along the coast of South Africa (insert) for which roman catches were reported by the boat-based commercial linefishery. Total landings of roman for the period 1985–2000 per 5 × 5 nautical mile grid cell are shown. ( b ) Goukamma area with boundaries of the MPA and access points (blue circles) for the local fishery. Grid cells where roman catches were reported are indicated. Full size image Generalized Additive Models (GAMs) with a delta-log-normal error distribution were used to standardize the CPUE time series of roman [14] in an area within 30 km from the boundary of the MPA. This area is consistent with the typical range of linefish vessels [11] and is likely to encapsulate the area of settlement of larvae originating from the MPA [6] , [15] , [16] ( Fig. 1b ). CPUE time series were also standardized in three other areas, together representing the entire remaining range of the species ( Fig. 1a ). In this article, we demonstrate that fisheries in the vicinity of MPAs can recover rapidly, possibly without negative consequences for fishers because of increased travel distances and reduction of catch rates. We conclude that this recovery is best explained by a succession of spillover of adult fish from the MPA followed by a recruitment boost caused by increased larval dispersal. Demonstrating a positive effect after the establishment of a MPA by analysing fishery data represents a significant step towards improving the acceptance of MPAs as a viable fishery management option. Trends in standardized CPUE Standardized CPUE before 1990 showed no trends throughout the roman fishery ( Fig. 2 ). After 1990, the CPUE in the vicinity of Goukamma MPA improved, eventually doubling the pre-reserve rate after 10 years ( Fig. 2c ). In all other areas, CPUE remained indistinguishable from the 1985 rates ( Fig. 2a,b,d ) with no discernible upward or downward trends. 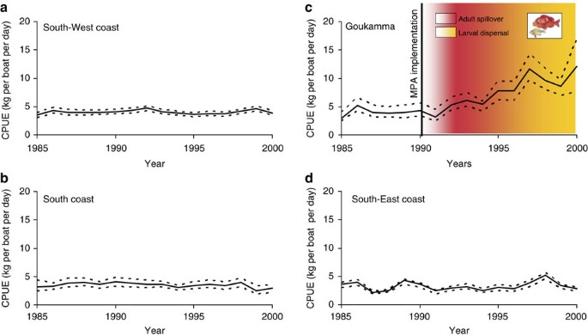Figure 2: Differences in CPUE between four coastal areas for the period 1985–2000. Standardized CPUE represented by solid trend lines with 95% confidence limits (broken lines). (a,b,d) No trends in CPUE detectable for the South-West coast, South coast and South-East coast areas. (c) Increasing CPUE for the Goukamma area after MPA implementation in 1990. Phases suggested to be attributed to adult spillover and larval dispersal are illustrated by red and yellow shading, respectively. Figure 2: Differences in CPUE between four coastal areas for the period 1985–2000. Standardized CPUE represented by solid trend lines with 95% confidence limits (broken lines). ( a , b , d ) No trends in CPUE detectable for the South-West coast, South coast and South-East coast areas. ( c ) Increasing CPUE for the Goukamma area after MPA implementation in 1990. Phases suggested to be attributed to adult spillover and larval dispersal are illustrated by red and yellow shading, respectively. Full size image Total catch and spatial distribution of fishing effort Total roman catch decreased from 1985 to 1991 in the Goukamma area, but started to increase 1 year after the MPA was implemented ( Fig. 3 ). It exceeded pre-reserve levels by 1996, in contrast to all other areas, where catches showed a general decline throughout the 16-year time series ( Fig. 3 ). At 5 × 5 nautical mile resolution, we found little systematic change in the spatial distribution of reef-directed fishing effort outside the MPA and no evidence for increased travel distance from the access points as a result of its declaration. Spatial information on roman-directed effort around Goukamma indicated that fishing was initially distributed within 15 nautical miles of the centre of the soon-to-be-declared MPA, and most effort was directed at reefs close to or inside its boundary ( Fig. 4a ). After the MPA implementation, effort remained concentrated at reefs in the same grid blocks close to the MPA borders ( Fig. 4b ), with little change over the 10 years of post-MPA observation ( Fig. 4c ). 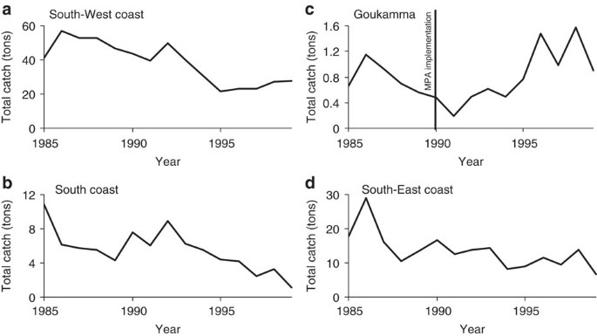Figure 3: Differences in commercial fishery catches between four coastal areas for the period 1985–2000. (a,b,d) Total catches generally declined in the South-West coast, South coast and South-East coast areas. (c) Total catch increased in the Goukamma area after MPA implementation in 1990. Figure 3: Differences in commercial fishery catches between four coastal areas for the period 1985–2000. ( a , b , d ) Total catches generally declined in the South-West coast, South coast and South-East coast areas. ( c ) Total catch increased in the Goukamma area after MPA implementation in 1990. 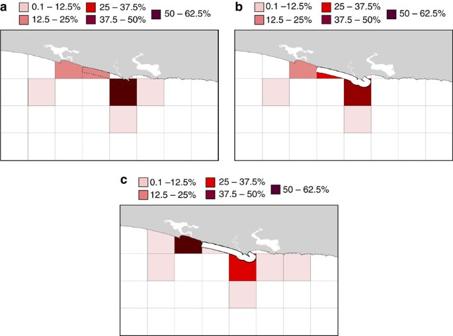Figure 4: Spatial patterns of reef fish directed effort for the Goukamma area for the period 1985–2000. Spatial patterns of the percentage of boat-based linefishing effort directed at reef fish for the periods of (a) 1985–1989, (b) 1990–1994 and (c) 1995–2000. Only negligible spatial changes were observed over the period. Full size image Figure 4: Spatial patterns of reef fish directed effort for the Goukamma area for the period 1985–2000. Spatial patterns of the percentage of boat-based linefishing effort directed at reef fish for the periods of ( a ) 1985–1989, ( b ) 1990–1994 and ( c ) 1995–2000. Only negligible spatial changes were observed over the period. Full size image The retrospective analysis of fishery-dependent data from South Africa suggests that the Goukamma MPA succeeded in achieving fishery management and conservation objectives. Roman is one of the several reef-dwelling predatory fish that have been heavily depleted by fishers [11] . Their characteristic features (high longevity, residency and broadcast spawning) are shared by temperate and tropical reef species throughout the world [17] , and MPAs have been shown to aid the recovery of depleted stocks of such species, but this is seldom sufficient to convince fishers and authorities to accept spatial closures as an integral part of fishery management [7] . It is postulated that a progression of two mechanisms, spillover and larval export from the MPA, best explains the trajectory of the increase in CPUE in the area around Goukamma ( Fig. 5 ). Spillover of adult roman should begin immediately at the onset of a density gradient across the MPA boundary. For species with density-independent movements, the rate of spillover and therefore the rate of CPUE increase outside the reserve should track this density gradient. Field studies of adult roman movements have shown that the species is resident, and that occasional home-range relocations are not density dependent [12] , [13] , [18] . However, the density gradient should stabilize once the biomass inside the MPA reaches an asymptote. The results of a spatially structured individual-based model based on life history data collected in and outside Goukamma [19] suggest that this asymptote should be reached 5 years after exploitation stops, as female roman abundance inside the MPA should recover to 100% and male abundance to 80% of pre-exploitation values, respectively. For this reason, CPUE increases observed after this period cannot be attributed to spillover alone. 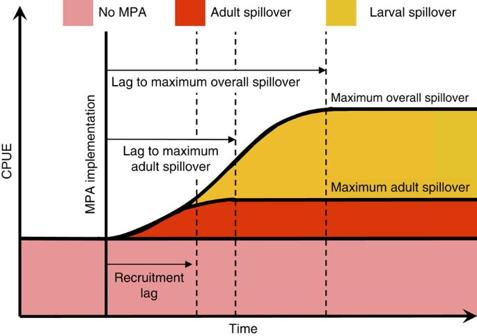Figure 5: Postulated mechanisms responsible for the increase of CPUE around MPAs. Spillover of adult fishes commences immediately with the growing density gradient between the MPA and the fished area, resulting in an increase in CPUE in the fished area, which reaches an asymptote when the biomass of adult fishes inside the MPA attains its maximum. The process is limited by the movement behaviour and the growth rate of the species, as well as by the distribution of suitable habitat across the MPA boundary. In contrast, larval export can only commence after the larvae spawned by the increasing population inside the MPA have settled and grown to recruitment size. The combined effect reaches its limit when maximum spawning capacity inside the MPA has been restored. Figure 5: Postulated mechanisms responsible for the increase of CPUE around MPAs. Spillover of adult fishes commences immediately with the growing density gradient between the MPA and the fished area, resulting in an increase in CPUE in the fished area, which reaches an asymptote when the biomass of adult fishes inside the MPA attains its maximum. The process is limited by the movement behaviour and the growth rate of the species, as well as by the distribution of suitable habitat across the MPA boundary. In contrast, larval export can only commence after the larvae spawned by the increasing population inside the MPA have settled and grown to recruitment size. The combined effect reaches its limit when maximum spawning capacity inside the MPA has been restored. Full size image A recruitment effect is needed to explain the sustained increase. Roman spawn throughout their range and their pelagic eggs and larvae are transported passively until the post-flexion larvae settle after about 17 days [10] . Current speeds at Goukamma are moderate [20] , but frequently change direction, and can retain larvae within the vicinity of the MPA [21] , [22] as shown for mussel larvae [22] . After a lag period corresponding to 5 years, the age-at-recruitment for roman [23] , the progeny from the unexploited cohorts in the reserve should start to become available to the fishery. In the case of sequential hermaphrodites such as roman, a collapsed population will have sperm limitation due to highly skewed sex ratios and severely decreased egg production capacity due to the paucity of large females. However, protected populations can recover rapidly [19] , resulting in a recruitment boost for the fishery within the range of larval export. The continued increase in CPUE after 1996 is consistent with this lag, and it suggests that the protection of roman in the MPA increased recruitment in the immediate surrounds. An economic argument against the use of MPAs as a fishery management tool is that they initially reduce catch [24] and could permanently increase the distance that fishers need to travel [25] . We found no evidence to suggest that the Goukamma MPA negatively affected fishers’ profits. The absence of any initial repercussions for fishers following the MPA implementation was surprising, but might be explained by the location of boat access points in relation to the MPA and the multi-species nature of the fishery, which is not reliant on reef fishes only. To our knowledge, this is one of a few studies that present empirical evidence of a fishery benefitting from a MPA without incurring additional costs, and the only one that attempts to separate the possible effects of spillover and larval dispersal by examining the temporal signature of each process within fishery data. In a recent global synthesis, fish abundance patterns around 14 reserves were evaluated with reaction-diffusion models to determine spillover and fishery compensation [26] . Although results were similar to this study, they were not derived from data covering periods before and after the establishment of the MPAs, and larval dispersal was not considered. Both these aspects have been investigated separately in the literature. For example, time-series fishery data from before and after reserve establishment around Apo Island were used to infer adult spillover [27] while genetic parental analyses revealed patterns of larval dispersal within a network of reserve sites on the Great Barrier Reef [16] . We were fortunate to have had a comprehensive spatially referenced catch-return data set from throughout the range of a fish species representing pre- and post-MPA conditions, combined with relative stability in fishing effort, but the characteristics of the fishery system investigated here are not unique. It could be expected that where MPAs have been established to protect depleted reef fishes, fisheries have benefitted in a similar manner. Time series of fisheries data might be available elsewhere to provide evidence for the mechanisms outlined here in other parts of the world, which might prove more convincing to fishers and decision makers than studies solely based on theoretical models. Information on the study species Roman is a seabream endemic to the warm-temperate South Coast of South Africa, where it feeds on invertebrates and fishes on rocky reefs to depths of 120 m. The species is a protogynous hermaphrodite, attains 19 years and matures at 3–4 years of age [23] . Adults are mainly resident within small home ranges of <100 m linear extent, but few individuals (~9%) travel distances over two magnitudes larger than the home range [12] , [13] . These movements are rapid, inconsistent in direction and independent of sex, size and fish density [12] , [13] . Roman spawn in the summer months throughout their range and their pelagic eggs and larvae are transported passively until they settle after about 17 days [10] . Roman consist of a single, well-mixed population [10] that has been exploited for over a century [11] . The population has been depleted to various degrees throughout its range, with minima of about 5% of historical abundance in many areas [11] . Diving and angling surveys in several MPAs, including Goukamma, indicate that roman respond well to spatial protection and abundance, size-structure, sex-ratio and age-at-sex-change have recovered inside reserves of all sizes [23] , [28] . Data selection The South African ‘linefishery’ operates almost exclusively from small, high-powered boats equipped with fishing rods or hand-lines along the entire South African coast. Catches include pelagic shoaling species, such as snoek ( Thyrsites atun ) and yellowtail ( Seriola lalandi ), and demersal species, such as kob ( Argyrosomus spp.) and geelbek ( Atractoscion aequidens ). The availability of these wide-ranging, shoaling species is erratic, and fishers consistently target reef-associated, high-value species such as roman. Since 1985, spatially referenced data on boat- and species-specific daily catch from the South African linefishery have been captured in the National Marine Linefish System hosted by the South African Department of Agriculture, Forestry and Fisheries, a relational database listed as one of the largest of its kind [29] . We considered data for the period from 1985 to 2000, covering the known distributional range of roman between Cape Point in the West and the Kei River in the East ( Fig. 1 ). After 2000, the depletion of many linefishes caused a drastic cut in linefish-directed effort, and the data were deemed not to be directly comparable. The raw data consist of vessel number, catch location referenced to a 5 × 5 nautical mile grid, catch in kilogram per species and catch date. First, the Goukamma area encompassing all grid cells that fell within a 30-km range from the MPA boundaries was isolated, equalling to an overall area of 14 grid cells alongshore and six grid cells offshore. This range was assumed to approximate the distance from the MPA in which increased abundance due to spillover and larval dispersal effects should be theoretically detectable [6] and also represents the range of the vessels that fish the Goukamma area from the three access points. In addition, the data set was subset into the three major reference biogeographical areas, namely the South-West coast, the South coast and the South-East coast ( Fig. 1 ). Only catch returns that reported reef fishes (see Supplementary Table S1 ) were included in our analyses to avoid inflation of ‘false’ zero catches caused by fishing trips that predominantly targeted non-reef-associated species. The number of vessels operating in the linefishery was highly variable, and vessels entered the fishery at different times throughout the study period. To select appropriate indicator vessels, unique vessel numbers were ranked according to the number of trips for which roman was reported and the number of years they operated in the fishery as a function of trips × years [2] . Of a total of 79 vessels that operated in the Goukamma area during the study period, we selected the first 15 vessels for CPUE standardization. These vessels reported over a period of at least 4 years during which they accounted for 56% of boat trips with reef fish landings and for 81% of the trips that landed roman (see Supplementary Table S2 ). For the three larger reference areas, we restricted our analysis to a maximum of 50 indicator vessels to avoid overparameterization. All grid cells with <200 records were excluded from data sets to minimize bias induced by isolated catch locations or inconsistencies in reporting. Statistical analysis of catch and effort data CPUE was assumed to be linearly proportional to abundance, as is common practice [14] , [30] , [31] , [32] . These fishery-dependent data introduce several challenges to the construction of reliable abundance indices because factors such as changes in spatial and temporal effort allocation, vessel effects or fishing behaviour need to be accounted for [14] , [30] , [31] , [32] , [33] , [34] . To standardize relative abundance indices for roman for the four areas, we applied GAMs with integrated smoothness estimation using penalized regression splines [35] for continuous predictor variables. All analyses were carried out within the ‘R’ statistical programming environment [36] and the ‘mgcv’ package [35] . As the CPUE data sets comprised relatively high proportions of zeros (23–57%) and positive CPUE values (CPUE pos ) were considerably right-skewed (see Supplementary Fig. S1 ), we assumed a two-stage delta-log-normal distribution to be an adequate statistical error model to account for the variability in the data [27] , [37] . Histograms of residuals and quantile–quantile plots indicated no violation of the log-normal error model for positive CPUE values (see Supplementary Fig. S2 ). This approach involves modelling the probability of zero catches and the quantity CPUE pos separately, which was realized by means of the following two sub-models: where logit denotes the link function of the logistic regression model that is used to predict the probability p of catching roman, ln(CPUE pos ) is the response of natural log-transformed positive CPUE values, s() denotes smoother functions (that is, cubic regression splines), and prop.reeffish denotes the proportion of reef-associated fish in the catch as a measure of targeted effort (see Supplementary Fig. S3 ). A bias-corrected natural estimate for the expected CPUE for the delta-log-normal model was then calculated as: where is the estimated model s.d. (residual s.e.) of the log-normal GAM. Final model selection was based on minimizing the Akaike Information Criterion values for each binomial and log-normal sub-model separately. The applied forward stepwise selection procedure resulted in the inclusion of all considered covariates for each sub-model of the four areas with a significant fraction of the total deviance explained by each predictor variable ( P <0.01, χ 2 -test; Supplementary Tables S3–S6 ). The total deviance explained in the binary data ranged from 15.8% for the South-East coast to 25.3% for the Goukamma area for the final binomial sub-models. The log-normal model components explained very similar percentages of the variation in the positive roman CPUE across the four areas, ranging between 39.0 and 40.4% (see Supplementary Tables S3–S6 ). Confidence intervals for expected yearly CPUE values were estimated by applying a non-parametric bootstrapping procedure [38] . The data set was re-sampled randomly with replacement, and both sub-models were executed 1,000 times. Confidence limits from resultant bootstrap vectors for the predicted year effect were obtained by applying the percentile method [39] , where the 2.5% and 97.5% percentiles were chosen to obtain the lower and upper 95% confidence intervals, respectively. How to cite this article: Kerwath, S. E. et al. Marine protected area improves yield without disadvantaging fishers. Nat. Commun. 4:2347 doi: 10.1038/ncomms3347 (2013).